PTPN2 attenuates T-cell lymphopenia-induced proliferation When the peripheral T-cell pool is depleted, T cells undergo homoeostatic expansion. This expansion is reliant on the recognition of self-antigens and/or cytokines, in particular interleukin-7. The T cell-intrinsic mechanisms that prevent excessive homoeostatic T-cell responses and consequent overt autoreactivity remain poorly defined. Here we show that protein tyrosine phosphatase N2 (PTPN2) is elevated in naive T cells leaving the thymus to restrict homoeostatic T-cell proliferation and prevent excess responses to self-antigens in the periphery. PTPN2-deficient CD8 + T cells undergo rapid lymphopenia-induced proliferation (LIP) when transferred into lymphopenic hosts and acquire the characteristics of antigen-experienced effector T cells. The enhanced LIP is attributed to elevated T-cell receptor-dependent, but not interleukin-7-dependent responses, results in a skewed T-cell receptor repertoire and the development of autoimmunity. Our results identify a major mechanism by which homoeostatic T-cell responses are tuned to prevent the development of autoimmune and inflammatory disorders. The capacity of naive T cells to respond to pathogens is dependent on T-cell receptor (TCR)-mediated recognition of foreign peptide antigens presented by major histocompatibility complex (MHC) molecules. However, the engagement of peptide antigen–MHC complexes is also required for T-cell development in the thymus, as well as T-cell homoeostasis in the periphery [1] , [2] . In the thymus, TCR interaction with self-peptide–MHC shapes the TCR repertoire; CD4 + CD8 + double-positive (DP) thymocytes with high-affinity TCRs that are capable of developing into autoreactive T cells undergo programmed cell death or ‘negative selection’, whereas those with low to moderate affinity for self-peptide–MHC undergo ‘positive selection’ and develop into CD4 + or CD8 + single positive (SP) thymocytes and thereon emigrate as mature T cells [1] , [2] . In the periphery, TCR interaction with self-peptide–MHC is essential for T-cell survival and homoeostasis. Moreover after acute T-cell depletion (lymphopenia), as occurs in response to insults such as severe stress, physical exertion, infection, radiation and chemotherapy, TCR-self-peptide–MHC interactions and the homoeostatic γc chain cytokines interleukin (IL)-7 and IL-15 drive cellular proliferation to replenish the T-cell pool [1] , [3] . Although endogenous ligands supporting lymphopenia-induced proliferation (LIP) remain to be identified, studies with TCR transgenic T cells indicate that the extent to which naive CD8 + T cells undergo LIP may be influenced by TCR affinity for peptide–MHC, so that T cells with higher affinity TCRs undergo faster LIP than T cells with lower affinity TCRs [1] , [4] , [5] , [6] , [7] . However, it remains unclear how T-cell responses to TCR-self-peptide–MHC interactions may be attenuated in the context of LIP to prevent overt autoreactivity and disease. Foxp3 + regulatory T cells can suppress the fast-paced form of LIP that can occur when naive T cells are transferred into immunocompromised Rag −/− or TCR α −/− mice [8] , [9] ; this fast-paced form of LIP is driven largely by the recognition of foreign gut antigens derived from the gut microflora [10] , [11] . Similarly, the need for co-stimulation by CD28 can also serve to restrict the fast-paced expansion of CD4 + T cells in Rag −/− mice [12] . However the extent to which such processes limit the LIP that is driven by the recognition of self-antigens under conditions of acute lymphopenia remains unknown. TCR ‘tuning’ may be an important process for the prevention of LIP-associated autoimmunity. TCR ‘tuning’ refers to the process wherein T-cell responses to self-antigens are suppressed by T cell-intrinsic mechanisms that develop before mature T cells leave the thymus [3] , [13] , [14] , [15] . Evidence for TCR tuning stems from studies comparing the responses of DP thymocytes and peripheral T cells to low-affinity peptides antigens; low-affinity antigenic peptides that are unable to activate mature effector cells can induce strong DP thymocyte deletion [16] . Several molecules that attenuate TCR signalling, including protein tyrosine phosphatases (PTPs), have been shown to be suppressed in DP thymocytes and upregulated in mature T cells and thus implicated in TCR tuning [3] , [13] . However, direct evidence that such negative regulators contribute to TCR tuning and serve to restrain T-cell responses in the context of LIP to prevent disease remains elusive. Genome-wide association studies have identified the PTP gene PTPN2 as an important non-MHC gene for autoimmunity [17] , [18] , [19] , [20] , [21] . Single nucleotide polymorphisms (SNPs) in PTPN2 have been linked with the development of Crohn’s disease, rheumatoid arthritis and type 1 diabetes [17] , [18] , [19] , [20] , [21] . At least one of the PTPN2 SNPs implicated in type 1 diabetes has been associated with a ~40% decrease in PTPN2 expression in T cells [22] . Recent studies have identified PTPN2 (also known as T-cell PTP; TCPTP) as a key regulator of TCR signalling in CD4 + and CD8 + T cells, serving to dephosphorylate and inactivate the Src family protein tyrosine kinases (SFK) Lck and Fyn that are instrumental in instigating TCR signalling [23] , [24] . PTPN2 has also previously been implicated in the dephosphorylation of Janus-activated kinases (JAK)-1/3 and several signal transducer and activator of transcription (STAT) family members for the attenuation of cytokine signalling [25] . T cell-specific PTPN2 deficiency enhances CD4 + and CD8 + T-cell responses in vivo and lowers the threshold for TCR-instigated responses so that CD8 + T cells respond more efficiently to peptide antigens with suboptimal TCR affinity [23] , [24] . Moreover, T cell-specific PTPN2-deficient mice ( Lck -Cre; Ptpn2 fl/fl ) develop widespread inflammation and spontaneous autoimmunity with age [23] , [24] , but the basis for this remains unclear. In this study we examine whether PTPN2 tunes T-cell responses to self in the context of LIP to prevent autoimmunity. We report that PTPN2 levels are increased in T cells leaving the thymus to attenuate TCR-dependent, but not cytokine-dependent LIP. Homozygous or heterozygous PTPN2 deficiency promotes a fast-paced T-cell LIP in irradiated mice commensurate with that occurring in response to commensal gut antigens in immunocompromised mice, alters the TCR repertoire and results in the development of autoimmunity. PTPN2 levels are increased in naive T cells To determine whether PTPN2 might tune TCR signalling to attenuate TCR responses to self-antigen in the periphery, we first compared PTPN2 protein levels in lymph node (LN)-naive CD4 + and CD8 + T cells to those in CD4 − CD8 − CD25 + double negative (DN), DP and CD4 + CD8 − and CD4 − CD8 + SP thymocytes. We assessed PTPN2 expression in thymocytes and T cells from C57BL/6 mice and from control ( Ptpn2 fl/+ ) versus T cell-specific PTPN2 heterozygous ( Lck -Cre; Ptpn2 fl/+ ) mice ( Fig. 1a–c ). We found that PTPN2 protein levels in thymocytes decreased as cells transitioned from the DN to DP stages and thereon increased in SP thymocytes and remained elevated in peripheral naive T cells ( Fig. 1a,b ). PTPN2 levels in DP thymocytes approximated those seen in Lck -Cre; Ptpn2 fl /+ SP thymocytes ( Fig. 1c ). The increase in PTPN2 protein levels in SP thymocytes and naive T cells versus DP thymocytes is consistent with a role in thymic selection [23] , [26] and the attenuation of T-cell responses to self in the periphery. 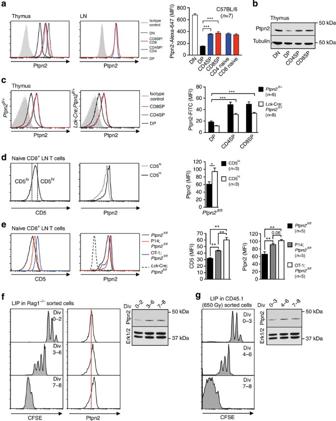Figure 1: AlteredPTPN2levels in thymocytes and T cells. (a,b) Thymocytes (DN: CD4−CD8−CD3loCD25hi; DP: CD4+CD8+CD3lo; CD4SP: CD4+CD8−CD3hi; CD8SP: CD4−CD8+CD3hi) and naive LN T cells from C57BL/6 mice and (c) thymocytes fromPtpn2fl/+versusLck-Cre;Ptpn2fl/+mice were either stained for PTPN2 (6F3) and analysed by flow cytometry or sorted and cell lysates resolved by SDS–PAGE and analysed by immunoblot analysis. (d) Naive LN T cells fromPtpn2fl/flwere stained for PTPN2 and CD5 and analysed by flow cytometry. (e) Naive LN T cells fromPtpn2fl/fl,Lck-Cre;Ptpn2fl/fl, P14;Ptpn2fl/fland OT- I;Ptpn2fl/flwere stained for PTPN2 and CD5 and analysed by flow cytometry. Naive CD8+LN T cells isolated from C57BL/6 (CD45.2+) mice were stained with CFSE and transferred into (f)Rag1−/−(CD45.1+) mice or (g) sub-lethally irradiated (650 Gy) CD45.1+mice. At 5 days and 10 days post transfer respectively, CD8+CD45.2+CFSE+splenic T cells were sorted for the indicated divisions (Div) and either stained for PTPN2 (6F3) and analysed by flow cytometry, or processed for immunoblot analysis. Where indicated PTPN2 mean fluorescence intensities (MFI) were determined; arbitrary units (a.u.) are shown. Representative flow cytometry profiles and quantified results (means±s.e.m.) for the indicated number of mice are shown. Results are representative of two (b,d–f) or three (a,c) independent experiments. Significance was determined using (a–c,e) two-tailed Mann–WhitneyU-test or (d) Student’st-test; *P<0.05, **P<0.01, ***P<0.001. Figure 1: Altered PTPN2 levels in thymocytes and T cells. ( a , b ) Thymocytes (DN: CD4 − CD8 − CD3 lo CD25 hi ; DP: CD4 + CD8 + CD3 lo ; CD4SP: CD4 + CD8 − CD3 hi ; CD8SP: CD4 − CD8 + CD3 hi ) and naive LN T cells from C57BL/6 mice and ( c ) thymocytes from Ptpn2 fl /+ versus Lck -Cre; Ptpn2 fl /+ mice were either stained for PTPN2 (6F3) and analysed by flow cytometry or sorted and cell lysates resolved by SDS–PAGE and analysed by immunoblot analysis. ( d ) Naive LN T cells from Ptpn2 fl/fl were stained for PTPN2 and CD5 and analysed by flow cytometry. ( e ) Naive LN T cells from Ptpn2 fl/fl , Lck -Cre; Ptpn2 fl / fl , P14; Ptpn2 fl/fl and OT- I; Ptpn2 fl/fl were stained for PTPN2 and CD5 and analysed by flow cytometry. Naive CD8 + LN T cells isolated from C57BL/6 (CD45.2 + ) mice were stained with CFSE and transferred into ( f ) Rag1 −/− (CD45.1 + ) mice or ( g ) sub-lethally irradiated (650 Gy) CD45.1 + mice. At 5 days and 10 days post transfer respectively, CD8 + CD45.2 + CFSE + splenic T cells were sorted for the indicated divisions (Div) and either stained for PTPN2 (6F3) and analysed by flow cytometry, or processed for immunoblot analysis. Where indicated PTPN2 mean fluorescence intensities (MFI) were determined; arbitrary units (a.u.) are shown. Representative flow cytometry profiles and quantified results (means±s.e.m.) for the indicated number of mice are shown. Results are representative of two ( b , d – f ) or three ( a , c ) independent experiments. Significance was determined using ( a – c , e ) two-tailed Mann–Whitney U -test or ( d ) Student’s t -test; * P <0.05, ** P <0.01, *** P <0.001. Full size image To further explore the concept of TCR tuning, we next correlated PTPN2 levels in naive (CD44 lo CD62L hi ) CD8 + T cells with CD5 expression; in polyclonal T cells, cell surface CD5 expression is directly proportional to the affinity of the TCR for self-peptide–MHC [27] , [28] . In keeping with a role in TCR tuning we found that PTPN2 was highest in polyclonal T cells with elevated CD5 ( Fig. 1d ). To further examine whether PTPN2 levels may be increased in T cells with high-affinity TCRs, we compared PTPN2 levels in polyclonal naive CD8 + T cells with those in naive OT-I (class I restricted TCR-specific for the ovalbumin peptide 257 SIINFEKL 264 (ref. 29 )) and P14 (class I restricted TCR specific for 33 KAVYNFATC 41 from gp33 lymphocytic choriomeningitis virus [30] ) T cells. CD5 levels were highest in OT-I CD8 + T cells, followed by P14 and then polyclonal CD8 + T cells ( Fig. 1e ). PTPN2 levels were also significantly higher in either P14 or OT-I T cells versus polyclonal T cells ( Fig. 1e ), consistent with a role in TCR tuning, but no significant differences were evident between P14 and OT-I T cells. Although PTPN2 may not differentially tune between these transgenic TCRs, these results are nonetheless consistent with PTPN2 tuning TCR signalling in a polyclonal T-cell pool. PTPN2 levels in T cells undergoing LIP Previous studies utilizing TCR transgenics have suggested that the extent to which naive T cells undergo LIP may be reliant on TCR affinity for peptide–MHC [1] , [4] , [5] , [6] , [7] . Accordingly, we asked whether PTPN2 levels may correlate with the extent of LIP, so that fast proliferating cells with higher affinity TCRs may have elevated PTPN2. CFSE-labelled naive CD8 + T cells were transferred into Rag1 −/− hosts, which completely lack T cells, and CFSE dilution was assessed after 5 days and correlated with PTPN2. In Rag1 −/− hosts, naive T cells undergo LIP that is reliant on TCR contact with peptide–MHC, but not cytokines [10] , [11] . We found that PTPN2 levels in CD8 + T cells (as monitored by flow cytometry or western blotting) reflected the extent of LIP, so that the highest PTPN2 levels were in the faster proliferating cells ( Fig. 1f ); similar results were obtained in CD8 + T cells undergoing LIP in irradiated hosts ( Fig. 1g ). To determine whether the varying PTPN2 levels may be indicative of TCR affinity, or a consequence of increased proliferation, we monitored for PTPN2 in CD8 + T cells that had undergone ex vivo proliferation in response to non-discriminatory TCR activation by crosslinking with α-CD3ε/α-CD28. PTPN2 levels were assessed over 4 days and after a varied number of divisions by immunoblot analysis. We found that PTPN2 levels were not altered by α-CD3ε/α-CD28-crosslinking irrespective of the duration of crosslinking, or the number of divisions ( Supplementary Fig. 1 ). Thus, TCR stimulation and proliferation per se are not sufficient to alter PTPN2 levels, consistent with the varying PTPN2 levels during LIP being T cell-intrinsic and reflecting TCR affinity. Taken together, these results indicate that PTPN2 may tune TCR signalling in the context of LIP to prevent excessive responses to self-antigens. PTPN2 deficiency enhances LIP To directly assess PTPN2’s role in TCR tuning and LIP we isolated naive (CD44 lo CD62L hi ) CD8 + T cells from control ( Ptpn2 fl/fl ) and T cell-specific PTPN2-deficient ( Lck -Cre; Ptpn2 fl/fl ) mice and labelled the cells with the fluorescent dye carboxyfluorescein diacetate succinimidyl ester (CFSE) to monitor T-cell expansion in vivo . CFSE-labelled cells were transferred into sub-lethally irradiated (to induce lymphopenia) congenic recipient mice and cell division assessed by the dilution of CFSE associated with cell division 3–7 days post transfer. We found that PTPN2 deficiency resulted in a significant increase in CD8 + T-cell proliferation in the spleens and livers of irradiated hosts ( Fig. 2a ; Supplementary Fig. 2a ). PTPN2-deficient CD8 + T cells undergoing LIP could be subdivided into ‘slow’ and ‘fast’ proliferating cells, with the latter constituting only a small fraction of the CFSE-labelled pool in mice receiving control Ptpn2 fl/fl CD8 + T cells. The proliferation of naive (CD25 lo CD44 lo CD62L hi ) CD4 + T cells in irradiated hosts was moderate after 7 days, with only ‘slow’ proliferating cells being evident ( Supplementary Fig. 2b ). Nonetheless, after more prolonged periods (21 days), both ‘fast’ and ‘slow’ proliferating CD4 + T cells were detected and this was exacerbated by PTPN2 deficiency ( Fig. 2b ). Control and PTPN2-deficient CD8 + T cells undergoing ‘slow’ proliferation expressed the cell surface marker CD62L, were intermediate for CD44 and low for CD49d ( Supplementary Fig. 3a ), consistent with these being antigen-inexperienced memory-phenotype T cells previously associated with T-cell homoeostasis and LIP [31] . On the other hand, roughly half of the rapidly proliferating CD8 + T cells acquired the characteristics of antigen-experienced effector (CD49d hi CD44 hi CD62L lo ) T cells [31] , [32] ; in the absence of PTPN2 a subset of these were KLRG1 hi consistent with them being terminally differentiated effector T cells ( Supplementary Fig. 3a ). Previously, we have reported that Lck -Cre; Ptpn2 fl/fl mice develop an effector/memory phenotype as early as 4 weeks of age that progressively develops over time [23] . The Lck -Cre; Ptpn2 fl/fl T cells arising from fast-paced LIP were phenotypically similar to those in 6-week old Lck -Cre; Ptpn2 fl/fl mice, wherein a proportion of the antigen-experienced activated T cells (CD49d hi CD44 hi CD62L lo ) were also IL7Rα lo KLRG1 hi ( Supplementary Fig. 3b ). These results indicate that PTPN2 deficiency promotes fast paced LIP and the acquisition of a terminal-effector phenotype. 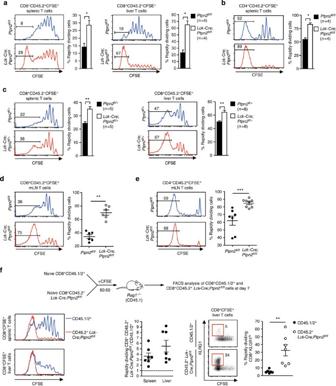Figure 2:PTPN2attenuates CD8+T-cell LIP. (a,b) Naive CD8+or CD4+LN T cells isolated fromPtpn2fl/flCD45.2+versusLck-Cre;Ptpn2fl/fl(CD45.2+) mice were stained with CFSE and transferred into sub-lethally irradiated (600 Gy) CD45.1+hosts. At 7-21 days post transfer splenic and liver T cells were analysed by flow cytometry. (c) CD8+naive T cells fromPtpn2fl/+(CD45.2+) andLck-Cre;Ptpn2fl/+(CD45.2+) mice were stained with CFSE and transferred into sub-lethally irradiated (650 Gy) CD45.1+hosts. At 8 days post transfer splenic and liver T cells were analysed by flow cytometry. (d,e) Naive CD8+or CD4+LN T cells fromPtpn2fl/flversusLck-Cre;Ptpn2fl/flwere stained with CFSE and transferred intoRag1−/−mice. At 7–10 days post transfer mesenteric LN (mLN) T cells were analysed by flow cytometry. (f) Naive CD8+LN T cells from CD45.1+/CD45.2+control mice and CD45.2+Lck-Cre;Ptpn2fl/flmice were stained with CFSE and co-transferred intoRag1−/−(CD45.1+) mice. At 7 days post transfer spleen and liver T cells were analysed by flow cytometry. In (a–f) representative CFSE profiles and quantified results (means±s.e.m.) are shown for the indicated number of mice. Results are representative of at least three independent experiments. Significance was determined using two-tailed Mann–WhitneyU-test; *P<0.05, **P<0.01, ***P<0.001. Figure 2: PTPN2 attenuates CD8 + T-cell LIP. ( a , b ) Naive CD8 + or CD4 + LN T cells isolated from Ptpn2 fl/fl CD45.2 + versus Lck -Cre; Ptpn2 fl/fl (CD45.2 + ) mice were stained with CFSE and transferred into sub-lethally irradiated (600 Gy) CD45.1 + hosts. At 7-21 days post transfer splenic and liver T cells were analysed by flow cytometry. ( c ) CD8 + naive T cells from Ptpn2 fl /+ (CD45.2 + ) and Lck -Cre; Ptpn2 fl /+ (CD45.2 + ) mice were stained with CFSE and transferred into sub-lethally irradiated (650 Gy) CD45.1 + hosts. At 8 days post transfer splenic and liver T cells were analysed by flow cytometry. ( d , e ) Naive CD8 + or CD4 + LN T cells from Ptpn2 fl/fl versus Lck -Cre; Ptpn2 fl/fl were stained with CFSE and transferred into Rag1 −/− mice. At 7–10 days post transfer mesenteric LN (mLN) T cells were analysed by flow cytometry. ( f ) Naive CD8 + LN T cells from CD45.1 + /CD45.2 + control mice and CD45.2 + Lck -Cre; Ptpn2 fl/fl mice were stained with CFSE and co-transferred into Rag1 −/− (CD45.1 + ) mice. At 7 days post transfer spleen and liver T cells were analysed by flow cytometry. In ( a – f ) representative CFSE profiles and quantified results (means±s.e.m.) are shown for the indicated number of mice. Results are representative of at least three independent experiments. Significance was determined using two-tailed Mann–Whitney U- test; * P <0.05, ** P <0.01, *** P <0.001. Full size image PTPN2 deficiency does not alter cytokine-mediated T-cell LIP Naive T-cell LIP is reliant on contact with self-peptide–MHC plus γc chain cytokines, especially IL-7 that signals via JAK1/3 and STAT5 (refs 1 , 33 , 34 ). On the other hand CD8 + memory T-cell (CD62L hi CD44 hi ) LIP is independent of contact with self-peptide–MHC and reliant on γc chain cytokines, especially IL-15 (refs 1 , 35 , 36 ). Since JAK1/3 and STAT5 can serve as PTPN2 substrates [37] , [38] , PTPN2 has the potential to regulate T-cell LIP, not only through the attenuation of TCR-SFK signalling [23] , [24] , but also through the attenuation of cytokine signalling. To assess the impact of PTPN2 deficiency on cytokine-induced CD8 + T-cell LIP, we first assessed responses in CD8 + (CD62L hi CD44 hi ) memory T cells. PTPN2 deficiency in memory CD8 + T cells resulted in enhanced TCR (α-CD3ε)-induced proliferation ex vivo ( Fig. 3a ). This is consistent with PTPN2 having the capacity to attenuate memory CD8 + TCR signalling and responses, as shown previously for naive CD8 + T cells [23] . However, in contrast to the promotion of naive CD8 + T-cell LIP ( Fig. 2a ), PTPN2 deficiency did not alter the proliferation of memory CD8 + T cells in irradiated hosts ( Fig. 3b ). The selective promotion of naive versus memory CD8 + T-cell LIP in irradiated mice suggests that the effects of PTPN2 deficiency on naive CD8 + T cells may be independent of cytokine signalling. Next, we directly assessed the impact on PTPN2 deficiency on IL-7 and IL-15 signalling. We found that IL-7-induced signalling in naive CD4 + or CD8 + T cells was not enhanced by PTPN2 deficiency; neither IL-7-induced JAK1 Y1022/Y1023 phosphorylation (pJAK1), nor overall STAT5 Y694 phosphorylation (pSTAT5) were increased by PTPN2 deficiency ( Fig. 4a–d ; Supplementary Fig. 4a ). Instead, at intermediate IL-7 doses, pSTAT5 was attenuated ( Fig. 4c,d ). Similarly, PTPN2 deficiency did not enhance IL-7-induced pSTAT5 in CD4 + and CD8 + memory T cells ( Fig. 3c ; Supplementary Fig. 4b ). Also, no overt differences were evident in IL-15-induced pSTAT5 in naive CD8 + T cells ( Fig. 4c ). However, IL-15-induced pSTAT5 signalling in naive CD4 + T cells and memory CD4 + T cells was significantly enhanced by PTPN2 deficiency ( Fig. 4d ; Supplementary Fig. 4b ). Interestingly, total STAT5, but not IL-7 receptor (CD127), IL-2/15 receptor (CD25/CD122), γc chain (CD132) or JAK1 levels were reduced by ~50–70% in PTPN2-null naive T cells ( Fig. 4e ; Supplementary Fig. 4c ). The decrease in STAT5 protein in naive T cells likely accounts for the reduced pSTAT5 evident at intermediate IL-7 doses ( Fig. 4c,d ). The decrease in STAT5 was not seen in the corresponding thymocytes ( Fig. 4e ), nor was it evident in heterozygous Lck -Cre; Ptpn2 fl /+ naive CD8 + T cells ( Supplementary Fig. 5 ). Importantly, heterozygous PTPN2 deficiency was sufficient to promote fast-paced CD8 + T-cell LIP in irradiated hosts ( Fig. 2c ), consistent with the enhanced Lck -Cre; Ptpn2 fl/fl naive CD8 + T-cell LIP being independent of alterations in STAT5. To explore this further and to exclude any possible influence of the environment in which Lck -Cre; Ptpn2 fl/fl T cells develop on the enhanced CD8 + T cell LIP, we assessed the impact of deleting PTPN2 in mature T cells. We bred PTPN2 floxed mice with Mx1 -Cre transgenic mice for the conditional deletion of PTPN2 in adult mice upon administration of poly (I:C). Using this approach we achieved ~80% PTPN2 deletion in naive CD8 + T cells; PTPN2 deletion in mature T cells did not alter STAT5 levels ( Fig. 4f ). We found that the proliferation of poly(I:C)-treated Mx1 -Cre; Ptpn2 fl/fl naive CD8 + T cells transferred to irradiated mice was significantly enhanced ( Fig. 4f ). Taken together these results are consistent with the enhanced naive CD8 + T-cell LIP being T cell-intrinsic and independent of γc chain cytokines and STAT5 signalling and the environment in which PTPN2-deficient T cells develop. 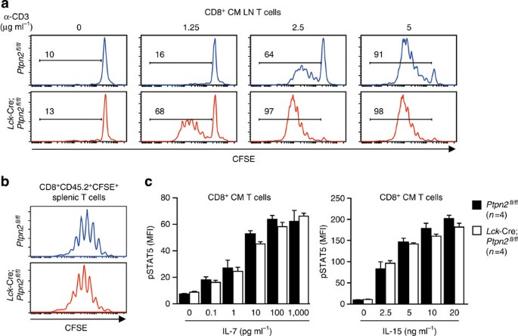Figure 3:PTPN2deficiency does not enhance CD8+CM T-cell LIP. (a) CD8+CM (CD8+CD62LhiCD44hi) LN T cells fromPtpn2fl/flversusLck-Cre;Ptpn2fl/flmice were stained with CFSE and stimulated with the indicated amounts of plate-bound α-CD3ε for 72 h and analysed by flow cytometry. (b) CD8+CM LN T cells fromPtpn2fl/fl(CD45.2+) andLck-Cre;Ptpn2fl/fl(CD45.2+) mice were stained with CFSE and transferred into sub-lethally irradiated (600 Gy) CD45.1+hosts. At 7 days post transfer splenic T cells were analysed by flow cytometry. (c) CD8+CM LN T cells fromPtpn2fl/flandLck-Cre;Ptpn2fl/flmice were stimulated with IL-7 or IL-15 for 15 min. Cells were stained for pSTAT5 and MFI determined by flow cytometry. In (a,b) representative CFSE profiles from two independent experiments are shown. Incquantified results are means±s.e.m. for the indicated number of mice and are representative of two independent experiments. Figure 3: PTPN2 deficiency does not enhance CD8 + CM T-cell LIP. ( a ) CD8 + CM (CD8 + CD62L hi CD44 hi ) LN T cells from Ptpn2 fl/fl versus Lck -Cre; Ptpn2 fl/fl mice were stained with CFSE and stimulated with the indicated amounts of plate-bound α-CD3ε for 72 h and analysed by flow cytometry. ( b ) CD8 + CM LN T cells from Ptpn2 fl/fl (CD45.2 + ) and Lck -Cre; Ptpn2 fl/fl (CD45.2 + ) mice were stained with CFSE and transferred into sub-lethally irradiated (600 Gy) CD45.1 + hosts. At 7 days post transfer splenic T cells were analysed by flow cytometry. ( c ) CD8 + CM LN T cells from Ptpn2 fl/fl and Lck -Cre; Ptpn2 fl/fl mice were stimulated with IL-7 or IL-15 for 15 min. Cells were stained for pSTAT5 and MFI determined by flow cytometry. In ( a , b ) representative CFSE profiles from two independent experiments are shown. In c quantified results are means±s.e.m. for the indicated number of mice and are representative of two independent experiments. 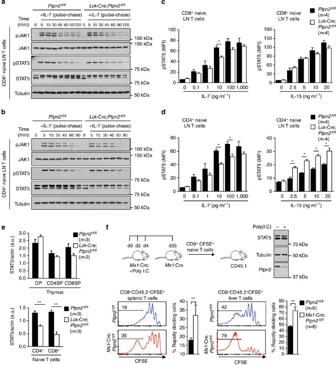Figure 4:PTPN2deficiency does not enhance cytokine signalling in CD8+T cells. (a) Naive CD8+or (b) CD4+LN T cells fromPtpn2fl/flandLck-Cre;Ptpn2fl/flmice were pulse-chased (5 ng ml−1, 10 min) with IL-7. Cell lysates were resolved by SDS–PAGE and immunoblotted as indicated. (c) Naive CD8+and (d) CD4+LN T cells fromPtpn2fl/flandLck-Cre;Ptpn2fl/flmice were stimulated with IL-7 or IL-15 for 15 min. Cells were stained for pSTAT5 and MFI determined by flow cytometry. (e) Cell lysates from DP, CD4SP and CD8SP thymocytes and naive CD4+and CD8+LN T cells isolated fromPtpn2fl/flandLck-Cre;Ptpn2fl/flmice were resolved by SDS–PAGE and immunoblotted for STAT5 and actin. STAT5 levels were quantified by densitometric analysis and normalised for actin. (f)Mx1-Cre;Ptpn2fl/flmice were injected with Poly (I:C) as indicated. PTPN2 and STAT5 levels inPtpn2fl/flCD8+naive T cells (−) and CD8+naive T cells from Poly (I:C)-treatedMx1- Cre;Ptpn2fl/flmice (+) were assessed by immunoblotting. CD8+naive T cells were isolated fromPtpn2fl/fl(CD45.2+) and Poly (I:C)-treatedMx1-Cre;Ptpn2fl/fl(CD45.2+) mice, stained with CFSE and transferred into sub-lethally irradiated (650 Gy) CD45.1+hosts. At 8 days post transfer splenic and liver T cells were analysed by flow cytometry. Representative immunoblots (a,b) and CFSE profiles (f) are shown. Quantified results are means±s.e.m. for the indicated number of mice and are representative of two (e,f) and at least three (a–d) independent experiments. Significance was determined using two-tailed Mann–WhitneyU-test; *P<0.05, **P<0.01. Full size image Figure 4: PTPN2 deficiency does not enhance cytokine signalling in CD8 + T cells. ( a ) Naive CD8 + or ( b ) CD4 + LN T cells from Ptpn2 fl/fl and Lck -Cre; Ptpn2 fl/fl mice were pulse-chased (5 ng ml −1 , 10 min) with IL-7. Cell lysates were resolved by SDS–PAGE and immunoblotted as indicated. ( c ) Naive CD8 + and ( d ) CD4 + LN T cells from Ptpn2 fl/fl and Lck -Cre; Ptpn2 fl/fl mice were stimulated with IL-7 or IL-15 for 15 min. Cells were stained for pSTAT5 and MFI determined by flow cytometry. ( e ) Cell lysates from DP, CD4SP and CD8SP thymocytes and naive CD4 + and CD8 + LN T cells isolated from Ptpn2 fl/fl and Lck -Cre; Ptpn2 fl/fl mice were resolved by SDS–PAGE and immunoblotted for STAT5 and actin. STAT5 levels were quantified by densitometric analysis and normalised for actin. ( f ) Mx1 -Cre; Ptpn2 fl/fl mice were injected with Poly (I:C) as indicated. PTPN2 and STAT5 levels in Ptpn2 fl/fl CD8 + naive T cells (−) and CD8 + naive T cells from Poly (I:C)-treated Mx1 - Cre; Ptpn2 fl/fl mice (+) were assessed by immunoblotting. CD8 + naive T cells were isolated from Ptpn2 fl/fl (CD45.2 + ) and Poly (I:C)-treated Mx1 -Cre; Ptpn2 fl/fl (CD45.2 + ) mice, stained with CFSE and transferred into sub-lethally irradiated (650 Gy) CD45.1 + hosts. At 8 days post transfer splenic and liver T cells were analysed by flow cytometry. Representative immunoblots ( a , b ) and CFSE profiles ( f ) are shown. Quantified results are means±s.e.m. for the indicated number of mice and are representative of two ( e , f ) and at least three ( a – d ) independent experiments. Significance was determined using two-tailed Mann–Whitney U -test; * P <0.05, ** P <0.01. Full size image PTPN2 deficiency enhances TCR-dependent LIP To examine whether the influence of PTPN2 deficiency on LIP is TCR-dependent, we first compared the responses of naive CD8 + T cells bearing the OT-I versus the P14 TCRs. PTPN2 deficiency significantly enhanced P14 T-cell LIP ( Fig. 5a ), albeit not as dramatically as that seen with polyclonal CD8 + T cells ( Fig. 2a ). On the other hand, PTPN2 deficiency had no effect on the proliferation of OT-I T cells in irradiated hosts ( Fig. 5a ). Moreover, neither wild type nor PTPN2-deficient OT-I or P14 T cells underwent the fast-paced LIP seen with polyclonal T cells ( Fig. 5a ). The lack of fast-paced LIP in T cells bearing transgenic TCRs has been reported previously, but the basis for this remains unclear [6] , [10] , [39] . Although OT-I T cells exhibited greater TCR affinity/avidity when compared with P14 T cells (as indicated by CD5 levels), there were no significant differences in PTPN2 levels ( Fig. 1e ). Thus, the lack of effect on OT-I T-cell LIP may be a consequence of the relatively high avidity of this TCR for self-peptide/MHC, which may override any effect of PTPN2 deficiency. Irrespective, the differential effects of PTPN2 deficiency on the ability of these two TCR transgenic T cells (and on polyclonal T cells) to undergo LIP is consistent with the impact of PTPN2 deficiency being TCR-dependent. 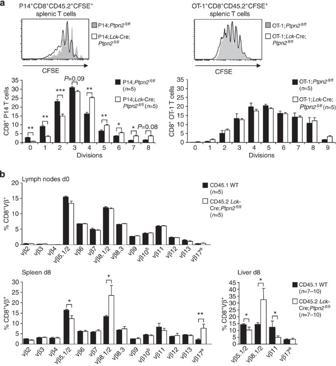Figure 5:PTPN2deficiency promotes TCR-dependent LIP and skews the TCR repertoire. (a) Naive CD8+LN T cells isolated from P14;Ptpn2fl/fl(CD45.2+) and P14;Lck-Cre;Ptpn2fl/fl(CD45.2+) or OT-1;Ptpn2fl/fl(CD45.2+) and OT-1;Lck-Cre;Ptpn2fl/fl(CD45.2+) were stained with CFSE and transferred into sub-lethally irradiated (650 Gy) CD45.1+hosts. At day 7 post transfer splenic T cells were analysed by flow cytometry. Representative CFSE profiles and quantified results are shown. (b) Naive CD8+LN T cells isolated from wild type (CD45.1+) andLck-Cre;Ptpn2fl/fl(CD45.2+) were pooled and transferred into sub-lethally irradiated (650 Gy) CD45.1+/CD45.2+hosts. At 8 days post transfer splenic and liver CD8+T cells were stained for the indicated TCRVβ-chains and analysed by flow cytometry. TCRVβ-chain frequencies before (d0) and after (d8) transfer are shown. Ina,bquantified results are means±s.e.m. for the indicated number of mice and are representative of at least three independent experiments. Significance was determined for (a) using one-way repeated measures ANOVA or (b) using two-tailed Mann–WhitneyU-test; *P<0.05, **P<0.01. Figure 5: PTPN2 deficiency promotes TCR-dependent LIP and skews the TCR repertoire. ( a ) Naive CD8 + LN T cells isolated from P14; Ptpn2 fl/fl (CD45.2 + ) and P14; Lck -Cre; Ptpn2 fl/fl (CD45.2 + ) or OT-1; Ptpn2 fl/fl (CD45.2 + ) and OT-1; Lck -Cre; Ptpn2 fl/fl (CD45.2 + ) were stained with CFSE and transferred into sub-lethally irradiated (650 Gy) CD45.1 + hosts. At day 7 post transfer splenic T cells were analysed by flow cytometry. Representative CFSE profiles and quantified results are shown. ( b ) Naive CD8 + LN T cells isolated from wild type (CD45.1 + ) and Lck -Cre; Ptpn2 fl/fl (CD45.2 + ) were pooled and transferred into sub-lethally irradiated (650 Gy) CD45.1 + /CD45.2 + hosts. At 8 days post transfer splenic and liver CD8 + T cells were stained for the indicated TCRVβ-chains and analysed by flow cytometry. TCRVβ-chain frequencies before (d0) and after (d8) transfer are shown. In a , b quantified results are means±s.e.m. for the indicated number of mice and are representative of at least three independent experiments. Significance was determined for ( a ) using one-way repeated measures ANOVA or ( b ) using two-tailed Mann–Whitney U- test; * P <0.05, ** P <0.01. Full size image If the effects of PTPN2 deficiency on T-cell LIP are influenced by TCR affinity, so that polyclonal T cells are variably expanded, then the resulting TCR repertoire should be skewed. To test this we assessed the TCR repertoire by comparing TCRVβ (Vβ2–14, Vβ17) usage in control (CD45.1 + ) and PTPN2-deficient (CD45.2 + ) naive CD8 + T cells before and after co-transfer into congenic irradiated hosts. Although no overt alteration in TCR usage was evident in CD8 + T cells from control versus PTPN2-deficient mice prior to transfer, we found that PTPN2-deficient LN, splenic and liver CD8 + T cells recovered 7 days post transfer exhibited a significant shift in TCRVβ usage ( Fig. 5b ; Supplementary Fig. 6 ). In particular, the frequency of PTPN2-deficient Vβ8.1/2 CD8 + T cells was increased and Vβ5.1/2 decreased in LNs, spleen and liver ( Fig. 5b ; Supplementary Fig. 6 ); the increase in Vβ8.1/2 cells was not due to an enrichment in NKT cells (as monitored with NK1.1; Supplementary Fig. 6a ). Moreover, an assessment of the resulting slow- and fast-proliferating wild type (CD45.1 + ) versus Lck -Cre; Ptpn2 fl/fl (CD45.2 + ) CD8 + T-cell pools in co-transfer experiments indicated that the alterations in TCRVβ usage reflected a greater proportion of PTPN2-deficient T cells being recruited to the fast proliferating pool, with overall T-cell numbers being unaltered ( Supplementary Fig. 7 ). Thus, PTPN2 deficiency variably promotes TCR-dependent LIP in a polyclonal T-cell pool to alter the TCR repertoire. To further explore PTPN2’s role in TCR-instigated responses, we next examined the impact of PTPN2 deficiency on the LIP that occurs under conditions of chronic lymphopenia. In hosts that completely lack T cells, such as mice lacking the recombination gene Rag1 , transferred CD4 + and CD8 + naive T cells can undergo fast-paced proliferation driven largely by peptide antigens from the gut microflora, rather than self-antigens [1] ; this fast-paced proliferation is reliant on TCR contact with peptide–MHC, but not cytokines [10] , [11] and results in the generation of antigen-experienced (CD49d hi ) effector/memory (CD44 hi CD62L lo ) T cells. To test the impact of PTPN2 deficiency on chronic LIP we transferred CFSE-labelled naive CD4 + or CD8 + T cells from Ptpn2 fl/fl or Lck -Cre; Ptpn2 fl/fl mice into Rag1 −/− mice and monitored proliferation in mesenteric LNs 10 days post transfer ( Fig. 2d,e ). Alternatively, CFSE-labelled naive CD8 + T cells from C57BL/6 (CD45.1 + /CD45.2 + ) and Lck -Cre; Ptpn2 fl/fl (CD45.2 + ) mice were co-transferred into Rag1 −/− (CD45.1 + ) mice and we monitored proliferation in liver and spleens 7 days post transfer ( Fig. 2f ). PTPN2 deficiency significantly enhanced the proliferation of CD8 + T cells in mesenteric LNs, spleen and liver in Rag1 −/− mice ( Fig. 2d,f ), with the last population being KLRG1 hi ( Fig. 2f ), consistent with these being terminally differentiated effector T cells. Moreover, in contrast to slow-paced CD4 + T-cell LIP evident in irradiated mice ( Fig. 2b ), naive CD4 + T cells underwent rapid expansion in Rag1 −/− mice and this was enhanced further by PTPN2 deficiency ( Fig. 2e ). Thus, TCR-mediated LIP under conditions of chronic lymphopenia is enhanced by PTPN2 deficiency. PTPN2 deficiency enhances responses to self- and gut antigens The enhanced T-cell LIP in Rag1 −/− mice raises the possibility that PTPN2 deficiency might enhance the response of T cells to commensal gut antigens even in irradiated mice. T-cell responses to gut antigens in irradiated mice are normally subdued by, amongst other things, the need for co-stimulation, the actions of regulatory T cells and possibly T-cell subsets that sustain the integrity of the gut wall [40] . However, the extent to which gut- versus self-antigens contribute to LIP in irradiated mice has not been formally examined. Previous studies have shown that fast-paced CD8 + T-cell LIP in Rag1 −/− mice can be largely prevented by antibiotic treatment and the eradication of the gut microflora [41] . To test whether the enhanced Lck -Cre; Ptpn2 fl/fl CD8 + T-cell LIP in irradiated mice is driven by self- versus commensal gut antigens, we treated recipient mice with a cocktail of antibiotics for two weeks, a condition that eliminated the gut microflora (as assessed by measuring bacterial 16S rRNA in faeces; Supplementary Fig. 8a ). Control and antibiotic-treated mice were then sub-lethally irradiated and Ptpn2 fl/fl or Lck -Cre; Ptpn2 fl/fl CFSE-labelled naive CD8 + T cells transferred for an assessment of LIP. We found that antibiotic treatment suppressed the fast-paced Ptpn2 fl/fl CD8 + T cell. LIP was evident in the liver, but not in the spleen, consistent with both gut- and self-antigens contributing to wild-type CD8 + T-cell LIP in irradiated mice ( Fig. 6 ; Supplementary Fig. 8b ). Importantly, antibiotic treatment ( Fig. 6 ; Supplementary Fig. 8b ) also suppressed but did not completely prevent the rapid Lck -Cre; Ptpn2 fl/fl CD8 + T-cell LIP in spleen and liver; Lck -Cre; Ptpn2 fl/fl CD8 + T-cell fast-paced LIP in antibiotic-treated mice continued to exceed that of Ptpn2 fl/fl CD8 + T cells in untreated controls ( Fig. 6 ). These results are consistent with PTPN2 deficiency enhancing CD8 + T-cell LIP induced by both gut- and self-antigens. Moreover, these results point towards PTPN2 deficiency enhancing CD8 + T-cell LIP to self-antigens in irradiated mice so that it is commensurate with that occurring in response to commensal gut antigens. 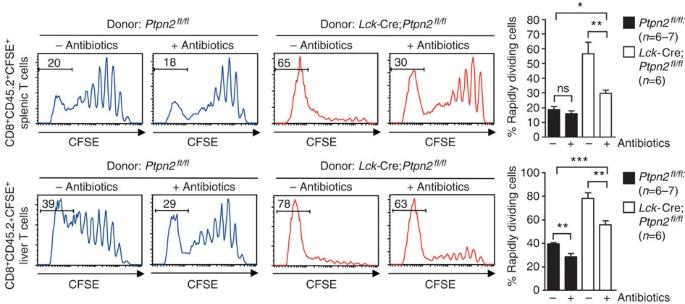Figure 6:PTPN2deficiency exacerbates CD8+T-cell responses to self- and gut antigens in irradiated mice. Naive CD8+LN T cells fromPtpn2fl/fl(CD45.2+) andLck-Cre;Ptpn2fl/fl(CD45.2+) were stained with CFSE and transferred into antibiotic-treated sub-lethally irradiated (650 Gy) CD45.1+hosts. At 8 days post transfer splenic and liver T cells were analysed by flow cytometry. Representative CFSE profiles and quantified results are shown. Quantified results are means±s.e.m. for the indicated number of mice and are representative of three independent experiments; significance was determined using two-tailed Mann–WhitneyU-test; *P<0.05, **P<0.01, ***P<0.001. Figure 6: PTPN2 deficiency exacerbates CD8 + T-cell responses to self- and gut antigens in irradiated mice. Naive CD8 + LN T cells from Ptpn2 fl/fl (CD45.2 + ) and Lck -Cre; Ptpn2 fl/fl (CD45.2 + ) were stained with CFSE and transferred into antibiotic-treated sub-lethally irradiated (650 Gy) CD45.1 + hosts. At 8 days post transfer splenic and liver T cells were analysed by flow cytometry. Representative CFSE profiles and quantified results are shown. Quantified results are means±s.e.m. for the indicated number of mice and are representative of three independent experiments; significance was determined using two-tailed Mann–Whitney U -test; * P <0.05, ** P <0.01, *** P <0.001. Full size image PTPN2-deficient LIP promotes disease A consequence of LIP and its proposed reliance on TCR affinity [1] , [4] , [5] , [6] , [7] is the preferential expansion of higher affinity T cells with decreased activation requirements and potentially increased risk for autoimmunity. We reasoned that by enhancing LIP to the level seen in response to foreign gut antigens and by skewing the TCR repertoire, PTPN2 deficiency might promote the development of autoimmunity. To test this we transferred Ptpn2 fl/fl versus Lck -Cre; Ptpn2 fl/fl naive CD8 + T cells into irradiated mice and assessed CD8 + T-cell subsets in blood and lymphoid tissues and monitored for the presence of lymphocytic infiltrates and tissue damage in non-lymphoid tissues such as liver and lung at 12–20 weeks post transfer. We found that PTPN2 deficiency resulted in the dramatic expansion of total and effector/memory (CD44 hi CD62L lo ) CD8 + T cells in blood and spleen and the infiltration of effector/memory T cells into liver and lung ( Fig. 7 ). The increase in hepatic lymphocytic infiltrates was accompanied by the development of liver damage, as assessed by the presence of the hepatic enzymes ALT (alanine transaminase) and AST (aspartate amino transferase) in serum, and was accompanied by high levels of anti-nuclear antibodies (ANA) in sera ( Fig. 7 ), indicative of a breakdown in tolerance. Importantly, albeit reduced, we found that enhanced LIP associated with heterozygous PTPN2 deficiency ( Fig. 2c ) was also accompanied by increased T-cell expansion, lymphocytic infiltrates in non-lymphoid tissues and signs of tissue damage and ANA in serum after 12–20 weeks ( Fig. 8 ; Supplementary Fig. 9 ), consistent with even a partial deficiency in PTPN2 being sufficient to abrogate PTPN2-mediated TCR tuning and contribute to the development of autoimmunity. Finally, to explore further the impact of PTPN2 deficiency in the promotion of LIP and disease we took advantage of Rag1 −/− that develop severe colitis after the transfer of naive T cells [41] . We transferred naive CD8 + T cells from Ptpn2 fl/fl versus Lck -Cre; Ptpn2 fl/fl mice with naive CD4 + T cells from C57BL/6 wild-type mice into Rag1 −/− mice and monitored for weight loss as an indicator of disease progression. We found that PTPN2 deficiency in CD8 + T cells promoted significant weight loss in Rag1 −/− mice ( Fig. 9a ), which was accompanied by colon distension and the enhanced expansion of CD8 + T cells without changes in CD4 + FoxP3 regulatory T (Treg) cells ( Fig. 9b,c ). Taken together these results are consistent with PTPN2 being instrumental in preventing excessive LIP and the development of autoimmune and inflammatory disease. 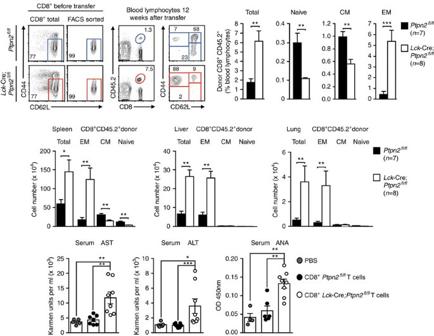Figure 7:PTPN2-deficient CD8+T cells promote autoimmunity in irradiated mice. Naive CD8+LN T cells fromPtpn2fl/fl(CD45.2+) versusLck-Cre;Ptpn2fl/fl(CD45.2+) mice were transferred into sub-lethally irradiated (600 Gy) CD45.1+hosts. At 12 weeks post transfer blood lymphocytes were analysed by flow cytometry. Relative numbers of total and naive (CD62LhiCD44lo), CM (CD62LhiCD44hi) and effector/memory (CD62LloCD44hi; EM) CD8+T cells were determined. Representative CD44 versus CD62L flow cytometry profiles before and after adoptive transfer are shown. At 20 weeks post transfer splenic, liver and lung lymphocytes were analysed by flow cytometry. Absolute numbers of total, naive, CM and EM CD8+T cells were determined. Serum ANA were measured and serum ALT and AST activities were determined. Results shown are means±s.e.m. for the indicated number of mice; significance was determined using a two-tailed Mann–WhitneyU-test; *P<0.05, **P<0.01, ***P<0.001. Figure 7: PTPN2- deficient CD8 + T cells promote autoimmunity in irradiated mice. Naive CD8 + LN T cells from Ptpn2 fl/fl (CD45.2 + ) versus Lck -Cre; Ptpn2 fl/fl (CD45.2 + ) mice were transferred into sub-lethally irradiated (600 Gy) CD45.1 + hosts. At 12 weeks post transfer blood lymphocytes were analysed by flow cytometry. Relative numbers of total and naive (CD62L hi CD44 lo ), CM (CD62L hi CD44 hi ) and effector/memory (CD62L lo CD44 hi ; EM) CD8 + T cells were determined. Representative CD44 versus CD62L flow cytometry profiles before and after adoptive transfer are shown. At 20 weeks post transfer splenic, liver and lung lymphocytes were analysed by flow cytometry. Absolute numbers of total, naive, CM and EM CD8 + T cells were determined. Serum ANA were measured and serum ALT and AST activities were determined. Results shown are means±s.e.m. for the indicated number of mice; significance was determined using a two-tailed Mann–Whitney U -test; * P <0.05, ** P <0.01, *** P <0.001. 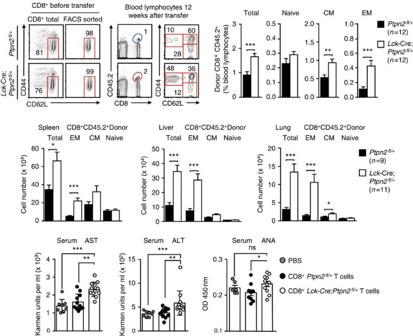Figure 8:Lck-Cre;Ptpn2fl/+PTPN2heterozygous CD8+T cells promote signs of autoimmunity in irradiated mice. Naive CD8+and CD4+LN T cells isolated fromPtpn2fl/+(CD45.2+) andLck-Cre;Ptpn2fl/+(CD45.2+) mice were co-transferred into sub-lethally irradiated (600 Gy) CD45.1+hosts. At 12 weeks post transfer blood lymphocytes were analysed by flow cytometry. Relative numbers of total, naive (CD62LhiCD44lo), CM (CD62LhiCD44hi) and effector/memory (CD62LloCD44hi; EM) CD8+T cells were determined. Representative CD44 versus CD62L plots before and after adoptive transfer are shown. At 20 weeks post transfer splenic, liver and lung lymphocytes were analysed by flow cytometry. Absolute numbers of total, naive, CM and EM CD8+T cells were determined. Serum ANA were measured and serum ALT and AST activities were determined. Results shown are means±s.e.m. for the indicated number of mice; significance was determined using a two-tailed Mann–WhitneyU-test; *P<0.05, **P<0.01, ***P<0.001. Full size image Figure 8: Lck-Cre;Ptpn2 fl/ + PTPN2 heterozygous CD8 + T cells promote signs of autoimmunity in irradiated mice. Naive CD8 + and CD4 + LN T cells isolated from Ptpn2 fl/ + (CD45.2 + ) and Lck -Cre; Ptpn2 fl /+ (CD45.2 + ) mice were co-transferred into sub-lethally irradiated (600 Gy) CD45.1 + hosts. At 12 weeks post transfer blood lymphocytes were analysed by flow cytometry. Relative numbers of total, naive (CD62L hi CD44 lo ), CM (CD62L hi CD44 hi ) and effector/memory (CD62L lo CD44 hi ; EM) CD8 + T cells were determined. Representative CD44 versus CD62L plots before and after adoptive transfer are shown. At 20 weeks post transfer splenic, liver and lung lymphocytes were analysed by flow cytometry. Absolute numbers of total, naive, CM and EM CD8 + T cells were determined. Serum ANA were measured and serum ALT and AST activities were determined. Results shown are means±s.e.m. for the indicated number of mice; significance was determined using a two-tailed Mann–Whitney U -test; * P <0.05, ** P <0.01, *** P <0.001. 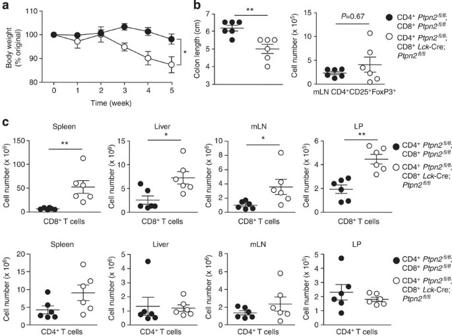Figure 9:PTPN2-deficient CD8+T cells exacerbate colitis inRag1−/−mice. Naive CD8+LN T cells fromPtpn2fl/flversusLck-Cre;Ptpn2fl/flmice were co-transferred with naivePtpn2fl/flCD4+T cells intoRag1−/−mice. (a) Colitis in recipientRag1−/−mice was assessed by body weight loss. (b,c) At 5 weeks post transfer recipient mice were killed and the colon removed and its length determined. The numbers of Foxp3+regulatory T cells in mLNs and CD8+and CD4+T-cell numbers in spleen, liver, mLNs and lamina propria were determined by flow cytometry. Quantified results are means±s.e.m. for the indicated number of mice and are representative of two different independent experiments; significance in (a) was determined using the two-way ANOVA test and in (b,c) using two-tailed Mann–WhitneyU-test; *P<0.05, **P<0.01. Full size image Figure 9: PTPN2- deficient CD8 + T cells exacerbate colitis in Rag1 −/− mice. Naive CD8 + LN T cells from Ptpn2 fl/fl versus Lck -Cre; Ptpn2 fl/fl mice were co-transferred with naive Ptpn2 fl/fl CD4 + T cells into Rag1 −/− mice. ( a ) Colitis in recipient Rag1 −/− mice was assessed by body weight loss. ( b , c ) At 5 weeks post transfer recipient mice were killed and the colon removed and its length determined. The numbers of Foxp3 + regulatory T cells in mLNs and CD8 + and CD4 + T-cell numbers in spleen, liver, mLNs and lamina propria were determined by flow cytometry. Quantified results are means±s.e.m. for the indicated number of mice and are representative of two different independent experiments; significance in ( a ) was determined using the two-way ANOVA test and in ( b , c ) using two-tailed Mann–Whitney U- test; * P <0.05, ** P <0.01. Full size image Recurrent lymphopenia may be an important factor in the development of autoimmunity. In humans several autoimmune diseases including type 1 diabetes, rheumatoid arthritis and Crohns have been associated with lymphopenia [42] , [43] . Moreover, mild lymphopenia and compensatory IL-21-dependent homoeostatic proliferation in nonobese diabetic mice that are prone to the development of autoimmunity have been reported to promote type 1 diabetes [44] , [45] . Similarly, deregulated regulatory T-cell expansion in lymphopenic nonobese diabetic hosts contributes to the development of type 1 diabetes [46] , whereas IL-7- mediated T-cell LIP in lupus or type 1 diabetes predisposed mice enhances their progression to disease [47] , [48] . In this study we have established for the first time the potential for excessive naive T-cell responses to peptide–MHC in the context of acute lymphopenia to alter the TCR repertoire and contribute to the development of autoimmunity. Our findings highlight the principal importance of PTPN2 in restraining naive T-cell responses to self- and/or gut antigens in the context of T-cell homoeostasis. We suggest that increases in PTPN2 in mature thymocytes and naive T cells may serve to limit TCR-mediated responses in the periphery during homoeostatic LIP to prevent autoimmunity. Importantly, our results indicate that the extent to which PTPN2 is increased in naive T cells may depend on TCR affinity. PTPN2 levels in naive CD8 + T cells correlated with CD5, a negative regulator of TCR signalling whose expression is considered to be indicative of TCR affinity [28] . PTPN2 levels were higher still in transgenic P14 and OT-I T cells; although self-ligands for the OT-I and P14 TCRs remain unknown, their proliferative responses and CD5 levels are consistent with them mediating higher avidity TCR responses. Moreover, PTPN2 levels in T cells undergoing LIP correlated with the rate of LIP, so that fast-paced cells expressed more PTPN2. Importantly, the elevated PTPN2 in fast-proliferating cells was not an outcome of stimulation or proliferation per se . Instead, we suggest PTPN2 levels may be instructed during thymic selection, so that PTPN2 is not only increased during the DP to SP transition, but that such increases correlate with TCR affinity. Thus, our results point towards PTPN2 tuning T-cell responses to antigen in the periphery for the maintenance of peripheral tolerance. Although PTPN2 has the capacity to regulate both TCR-mediated signalling, through the dephosphorylation of SFKs [23] , [49] , [50] , and IL-7/IL-15-mediated signalling, through the dephosphorylation of JAK1/3 and STAT5 (refs 37 , 38 ), our studies are consistent with the effects of PTPN2 deficiency on CD8 + T-cell LIP at least being independent of cytokine signalling, since (1) IL-7 signalling was not enhanced by PTPN2 deficiency in naive T cells, (2) IL-7/IL-15 signalling was not enhanced by PTPN2 deficiency in memory T cells, (3) PTPN2 deficiency did not alter CD8 + memory T cell LIP and (4) PTPN2 deficiency did not alter OT-I CD8 + naive T-cell LIP, despite OT-I T cells being reliant on IL-7 (ref. 51 ). However, since STAT5 levels were decreased, but IL-7-induced p-STAT5 was largely unaltered in naive PTPN2-deficient T cells, our results do not preclude PTPN2 deficiency otherwise promoting IL-7 signalling and LIP in naive T cells. Moreover, although IL-15 is not required for naive CD4 + T-cell LIP (ref. 51 ), the enhanced IL-15 signalling in PTPN2-deficient CD4 + may nonetheless contribute. Interestingly, humans bearing the rs1893217 SNP in PTPN2 exhibit reduced IL-2/IL-15-induced p-STAT5 in memory CD4 + T cells, without changes in total STAT5 (ref. 22 ). In mice, IL-15-induced pSTAT5 signalling was enhanced by PTPN2 deficiency in CD4 + memory T cells. Although PTPN2 function in memory T cells may be different in humans, it is also possible that decreased pSTAT5 in human CD4 + memory T cells may be an outcome of extrinsic cues. In keeping with PTPN2 regulating TCR-dependent LIP, we found that PTPN2 deficiency altered the TCR repertoire in polyclonal CD8 + T cells that had undergone LIP in irradiated hosts. Moreover, PTPN2 deficiency enhanced LIP for P14, but not OT-I TCR transgenic T cells. Why did PTPN2 deficiency not affect OT-I T-cell LIP? As discussed, PTPN2 levels in polyclonal T cells correlated with TCR affinity for self-antigen (as reflected by CD5) and the rate of LIP. In contrast, PTPN2 levels were not enhanced in OT-I T cells when compared with P14 T cells, despite OT-I TCR avidity (as reflected by CD5) being greater than that of P14. These results suggest that a threshold in TCR affinity may exist, beyond which PTPN2 may no longer tune, and PTPN2 deficiency may no longer affect TCR-instigated responses. This is in keeping with previous studies from our laboratory demonstrating that PTPN2 sets the threshold for TCR-instigated responses, so that PTPN2 deficiency minimally affects the proliferative responses of higher avidity TCRs (such as the OT-I TCR) engaging cognate peptide antigen [23] . It is possible that for very high-affinity TCRs, other PTPs may contribute to TCR tuning. For example, SHP-1/PTPN6, which interacts with CD5 to attenuate TCR signalling [52] , may be elevated to limit the impact of PTPN2 deficiency on LIP in OT-I T cells. In keeping with this, recent studies have shown that SHP-1 levels coincide with TCR affinity in CD8 + T cells [53] . Nonetheless, the selective effects of PTPN2 deficiency on P14 versus OT-1 T cells and the discrete alterations in the TCR repertoire point towards PTPN2 exerting preferential effects on a subset of T cells to promote their expansion. Since PTPN2 levels in thymocytes declined as cells transitioned from the DN to DP stages and increased again in SP thymocytes, these results are consistent with PTPN2 also having a role in establishing central tolerance and regulating thymocyte selection. In keeping with this we have reported previously that homozygous PTPN2 deficiency in thymocytes enhances both positive selection and negative selection [23] , [26] . At this stage the basis for the altered PTPN2 levels during thymocyte development remain unclear. In recent years the roles of microRNAs (miRNAs) in T-cell development and CD8 + T-cell responses have gained considerable attention [13] , [54] , [55] , [56] . In particular, it has been established that miRNA-181a expression during thymocyte development is low in DN4 thymocytes, increases in DP thymocytes and then decreases again in SP thymocytes and naive T cells [13] . Moreover, increases in miRNA-181a augment TCR signalling and T-cell responses by suppressing the expression of the phosphatases SHP-2/PTPN11 , PTPN22 and DUSP6 that function collectively to affect T-cell sensitivity [13] . Since miRNA-181a expression mirrors that of PTPN2 it is possible that PTPN2 may also be a target of miRNA-181a. Another possibility is that PTPN2 levels may be affected by extrinsic cues such as growth factors and cytokines. Transforming growth factor β (TGFβ) has been shown to attenuate naive T-cell responses to low-affinity antigens and to repress the rapid expansion and differentiation of T cells under conditions of acute or chronic lymphopenia [57] . Interestingly, recent studies have shown that TGFβ can upregulate the expression of miRNA-181a in metastatic breast cancer cells [58] . Our studies demonstrate that heterozygous PTPN2 deficiency in naive CD8 + T cells is sufficient to augment CD8 + T-cell LIP in irradiated hosts. Considering that PTPN2 levels in Lck -Cre; Ptpn2 lox /+ SP thymocytes and naive T cells approximated those in Ptpn2lox/lox DP thymocytes, these results point towards even a 50% decrease in PTPN2 being sufficient to counter the effects of the elevated phosphatase on TCR tuning. In keeping with this we found that the expansion of Lck -Cre; Ptpn2 lox /+ T cells in lymphopenic hosts was accompanied by signs of autoimmunity. Therefore, the findings of this study provide key insights into the molecular and cellular mechanisms by which PTPN2 SNPs, at least in naive CD8 + T cells, can contribute to the development of autoimmune diseases, such as type 1 diabetes [17] , [18] , [19] , [20] . Moreover, given the enhanced naive CD4 + and CD8 + T-cell LIP and the promotion of colitis in Rag1 −/− mice, our studies also reveal how PTPN2 SNPs can exacerbate responses to gut antigens and contribute to the development of inflammatory bowel diseases such as Crohns [18] , [19] , [21] . Hence, our studies identify an important non-MHC-dependent and T cell-intrinsic mechanism for the establishment of tolerance to self- and gut antigens and the prevention of autoimmune and inflammatory diseases. Mice All experiments were performed in accordance with the NHMRC Australian Code of Practice for the Care and Use of Animals. All protocols were approved by the Monash University School of Biomedical Sciences Animal Ethics Committee (ethics number: BAM/B/2005/38; MARP/2012/124). Ptpn2 fl/fl (C57BL6), Lck -Cre; Ptpn2 fl/fl (C57BL6), Mx1 -Cre; Ptpn2 fl/fl (C57BL6) and the corresponding OT-1 and P14 TCR transgenic mice as well as B6.SJL-Ptprc a Pep3 b /BoyJArc (Ly5.1/CD45.1), B6.SJL-Ptprc a Pep3 b /BoyJArc (Ly5.1/Ly5.2), B6.129S7-Rag1 tm1Mom /J ( Rag1 −/− ) mice on the Ly5.1/CD45.1 background and B6.129S7-Rag1 tm1Mom /Arc ( Rag1 −/− ) on the Ly5.2/CD45.2 background mice were maintained on a 12 h light–dark cycle in a temperature-controlled high barrier facility with free access to food and water. For adoptive transfers, 6–8-week-old female recipient mice and 3–6-week-old male or female donor mice were used. Exclusively female donor cells were used for transfers into female B6.129S7-Rag1 tm1Mom /ARC mice. For ex vivo experiments either male or female mice were used; Ptpn2 fl/fl and Lck -Cre; Ptpn2 fl/fl mice were sex-matched. Ptpn2 fl/fl and Lck -Cre; Ptpn2 fl/fl mice and the corresponding OT-I TCR transgenic mice were described previously [23] . Ly5.1/CD45.1 and B6.129S7-Rag1 tm1Mom /Arc ( Rag1 −/− ) mice on the Ly5.2/CD45.2 background were purchased from the Animal Resources Centre (Perth, Australia) and B6.129S7-Rag1 tm1Mom /J ( Rag1 −/− ) mice on the Ly5.1/CD45.1 background were purchased from WEHI Animal Facility (Kew, Australia). P14 TCR transgenic mice [30] were a gift from Scott Mueller (University of Melbourne, Australia) and Mx1 -Cre mice [59] were a gift from Carl Walkley (St Vincent’s Institute, Australia). Materials Mouse α-phospho-STAT5 (Y694) (14H2), rabbit α-phospho-JAK1 (Y1022), rabbit α-STAT5 (3H7) and rabbit α-JAK1 were purchased from Cell Signalling Technology; α-actin (sc-1616) was from Santa Cruz; hamster α-mouse CD3ε (145-2C11) and α-mouse CD28ε (145-2C11) from BD Biosciences and mouse α-tubulin (Ab-5) from Sigma-Aldrich. All antibodies were used at a dilution of 1/1,000 for immunoblotting with the exception of α-actin and α-tubulin that were used at dilutions of 1/2,000 and 1/5,000, respectively. Polyinosinic–polycytidylic acid sodium salt (poly (I:C)), Percoll and Dnase I were purchased from Sigma-Aldrich; fetal bovine serum (HyClone) from Thermo Scientific and Dulbecco-phosphate buffered saline (D-PBS) and Hank’s buffered salt solution (HBSS) from Invitrogen. Collagenase D was from Roche; the mouse ANA Ig’s (total IgA+G+M) ELISA Kit from Alpha Diagnostic International and the Transaminase CII kit from Wako Pure Chemical. The genomic DNA stool isolation kit was purchased from Qiagen. Rat α-CD16/CD32 (2.4G2) hybridoma supernatant was a gift from D.I. Godfrey (University of Melbourne, Australia), while the mouse α-PTPN2 (6F3) hybridoma supernatant was provided by Michel Tremblay (McGill University, Canada). Flow cytometry Lymphocytes from freshly dissected thymi, spleens, LNs, lungs and livers were isolated and processed for flow cytometry as described previously [23] . Red blood cells contaminating lymphocytes obtained from spleen, lung and liver were lysed using a 0.17 M hypotonic ammonium chloride buffer. Cells (1 × 10 6 per 10 μl) were resuspended in D-PBS/2% FBS and stained in 96-well microtitre plates (Falcon, BD Biosciences) for 20 min at 4 °C. For sorting, cells were stained in 15 ml Falcon tubes (BD Biosciences) for 30 min at 4 °C. Cells were washed and resuspended in D-PBS/2% FBS and data were collected using a LSRII (BD Biosciences) or CyAn ADP (Beckman Coulter) flow cytometer. Data were analysed using FlowJo7 (Tree Star Inc.) software. For cell sorting Influx (BD Biosciences) sorters were used. The following antibodies from BD Pharmingen (San Jose, CA, USA) were used for staining: 0.2 μg ml −1 fluorescein-isothiocyanate (FITC)-conjugated or phycoerythrin (PE)-cyanine dye 5 (Cy5)-conjugated or BD Horizon V450-conjugated α-CD44 (IM7), 0.2 μg ml −1 PE-conjugated or allophycocyanin (APC)-conjugated α-CD62L (MEL-14), 0.2 μg ml −1 Horizon PE-CF594-conjugated or Alexa Fluor 647-conjugated α-CD8 (53-6.7), 0.2 μg ml −1 PE-conjugated or PE-cyanine dye 7 (Cy7)-conjugated α-CD4 (RM4-5), 1 μg ml −1 PE-conjugated α-CD5 (53-7.3), PE-conjugated NK1.1 (PK136), 5 μg ml −1 FITC-conjugated α-TCRVβ2 (B20.6), -Vβ3 (KJ25), -Vβ4 (KT4), -Vβ5.1/5.2 (MR9-4), -Vβ6 (RR4-7), -Vβ7 (TR310), -Vβ8.1/8.2 (MR5-2), -Vβ8.3 (1B3.3), -Vβ9 (MR10-2), -Vβ10 b (B21.5), -Vβ11 (RR3-15), -Vβ12 (MR11-1), -Vβ13 (MR12-3) and -Vβ17 a (KJ23), 0.25 μg ml −1 APC-conjugated α-KLRG1 (2F1), 0.5 μg ml −1 PE-Cy7-conjugated α-CD45.1 (A20), 0.5 μg ml −1 PE-conjugated or Pacific Blue-conjugated α-CD45.2 (104), 1.25 μg ml −1 biotinylated α-CD49d (R1-2), 0.5 μg ml −1 APC-conjugated or PE-conjugated α-CD25 (PC61), 2 μg ml −1 PE-conjugated α-CD122 (TM-β1), 2 μg ml −1 PE-conjugated α-CD127 (SB/199), 2 μg ml −1 PE-conjugated α-CD132 (4G3) and 0.25 μg ml −1 V500-conjugated streptavidin. Pacific Blue-conjugated α-CD8 (5H10) used at 0.2 μg ml −1 was purchased from Invitrogen (Invitrogen-Molecular Probes, Carlsbad, CA, USA) or BioLegend (San Diego, CA, USA) and Pacific Blue-conjugated α-FoxP3 used at 1 μg ml −1 was purchased from eBioscience (San Diego, CA, USA). Cytokine signalling About 1–2 × 10 7 FACS-purified naive CD4 + and CD8 + CD62L hi CD44 lo T cells were stimulated with 5 ng ml −1 murine IL-7 (Peprotech) for 15 min at 37 °C. After stimulation cells were washed and resuspended in RPMI/1% FBS. Cells were incubated for the indicated times at 37 °C in the absence of murine IL-7 and lysed in modified RIPA buffer (50 mM Hepes (pH 7.4), 1% ( v / v ) Triton X-100, 1% ( v / v ) sodium deoxycholate, 0.1% ( v / v ) SDS, 150 mM NaCl, 10% ( v / v ) glycerol, 1.5 mM MgCl2, 1 mM EGTA, 50 mM NaF, leupeptin (5 mg ml −1 ), pepstatin A (1 mg ml −1 ), aprotinin (1 mg ml −1 ), 1 mM benzamidine, 2 mM phenylmethylsulfonyl fluoride, 1 mM sodium vanadate) and processed for immunoblotting using the specified antibodies. Uncropped blots have been provided in Supplementary Figure S10 . Intracellular staining Thymocytes/T cell (5 × 10 6 ) were fixed in 2 ml of 2% paraformaldehyde for 10 min at room temperature followed by a single wash with D-PBS. Cells were permeabilized in 1 ml methanol/acetone (50:50) for 30 min on ice and washed three times with D-PBS/5% FBS and processed for intracellular staining with either mouse α-PTPN2 (6F3) at a dilution of 1/100 or rabbit α-phospho-STAT5 (Y694) (D47E7; Cell Signalling Technology) at a dilution of 1/200 in D-PBS/5% FBS for 1 h at room temperature. Prior to PTPN2 staining cells were incubated for 20 min at room temperature with α-CD16/CD32 (1/50 dilution) to block Fc-receptors. Mouse IgG (H+L), F(ab′)2 fragment-FITC (1:200 dilution) or -Alexa 647 (1/800 dilution; Molecular Probes, Invitrogen) were used as secondary antibodies for PTPN2 staining, whereas for phosphorylated STAT5, rabbit IgG (H+L), F(ab′)2 fragment DyLight 649 (Jackson ImmunoResearch) was used at a dilution of 1:800. Cells were then incubated in 10% ( v / v ) rabbit serum or 10% ( v / v ) mouse serum (Invitrogen) to block unsaturated binding sites followed by staining for surface markers as described previously [23] . For the intracellular staining of CD4 + CD25 + FoxP3 + regulatory T cells the Foxp3/Transcription Factor Staining Buffer Set (eBiosciences) was used according to the manufacturer’s instructions. Naive and memory T-cell purification Naive and central-memory (CM) CD4 + and CD8 + T cells used for adoptive transfer experiments and proliferation assays were isolated from pooled peripheral LNs and purified by FACS with an Influx Sorter (BD Biosciences) to obtain naive CD62L hi CD44 lo or CD62L lo CD44 hi CM T cells. CD4 + CD8 + , CD4 − CD8 + or CD4 + CD8 − thymocytes were also purified by FACS. Sorted naive CD62L hi CD44 lo CD4 + and CD8 + T cells and CD4 + CD8 + thymocytes were routinely tested for purity (>99%). The purity for FACS purified CD4 + CD8 + and CD4–CD8 + thymocytes was >95%. In vitro T-cell proliferation For an assessment of T-cell proliferation in vitro FACS-purified T lymphocytes (1–5 × 10 7 per ml) were incubated in D-PBS supplemented with 0.1% ( v / v ) BSA containing 2–5 μM CFSE (Invitrogen, Molecular Probes) for 5 min at room temperature. Cells were then washed three times with PBS supplemented with 10% ( v / v ) FBS and stimulated with plate bound α-CD3ε (0–10 μg ml −1 ) in complete RPMI medium (RPMI 1640 (Invitrogen) supplemented with 10% ( v / v ) heat-inactivated FBS (HyClone, Thermo Scientific), 1 × non-essential amino acids (Sigma-Aldrich), 1 mM sodium pyruvate (Sigma-Aldrich), 2 mM L-glutamine (Invitrogen), 50 mM β-mercaptoethanol (Sigma-Aldrich) plus 100 U ml −1 penicillin and 100 mg ml −1 streptomycin incubated at 37 °C, 5% CO2, for 72 h. LIP and adoptive transfers Recipient CD45.1 + or CD45.1 + /CD45.2 + mice were sub-lethally irradiated with 600–650 Gy 24 h before adoptive transfer. Mice received aliquots of 0.25–2 × 10 6 sorted CD4 + or CD8 + naive or CM LN T cells stained with 5 μM CFSE in 100 μl sterile D-PBS by intravenous injection. At day 7 or 8 post transfer spleen, LN and liver lymphocytes of recipient mice were stained with fluorochrome-conjugated α-CD8 or α-CD4 and α-CD45.2 or α-CD45.1/2 and analysed by flow cytometry. Polyinosinic–polycytidylic acid treatment Mx1 -Cre; Ptpn2 fl/fl mice were injected intraperitoneally with 250 μg polyinosinic–polycytidylic acid (Poly (I:C)) in D-PBS every other day over 5 days. At day 35 mice were killed, naive LN CD8 + CD62L hi CD44 lo T cells isolated, stained with CFSE and transferred into sub-lethally irradiated (650 cGy) CD45.1 + mice. At day 8 post transfer spleen and liver lymphocytes were stained with fluorochrome-conjugated α-CD8 and α-CD45.2 and analysed by flow cytometry. Colitis model Recipient Rag1 −/− mice received sorted CD4 + (7.5 × 10 5 ) and CD8 + (7.5 × 10 5 ) naive LN T cells in 100 μl sterile D-PBS by intravenous injection. Body weights were monitored on a weekly basis using an analytical balance. At week 5 post transfer spleen, mesenteric LN (mLN), liver and lamina propria lymphocytes were stained with fluorochrome- conjugated α-CD4, α-CD8, α-CD44 and α-CD62L and analysed by flow cytometry. For the isolation of lamina propria lymphocytes the colon was cut into 0.5–1 cm pieces and incubated twice with Ca 2+ - and Mg 2+ -free HBSS supplemented with 5% ( v / v ) FBS, 2 mM EDTA, 0.15 mg ml −1 DTT and 10 mM Hepes shaking at 250 r.p.m. for 15 min at 37 °C to remove intra-epithelial lymphocytes and epithelial cells. Intestine pieces were digested in Ca 2+ - and Mg 2+ -containing HBSS supplemented with 5% ( v / v ) FBS, 1.5 mg ml −1 Collagenase D and 0.02 mg ml −1 Dnase I shaking at 250 r.p.m. for 1 h at 37 °C. Lymphocytes from digested tissue were enriched using a two-layer Percoll gradient at 40 and 80% ( v / v ) in DMEM supplemented with 10% ( v / v ) FBS. Antibiotic treatments CD45.1 + mice received drinking water containing 1 g l −1 ampicillin sodium (Aspen), 1 g l −1 metronidazole (Sanofi Aventis), 1 g l −1 neomycin sulphate (Jurox) and 500 mg l −1 vancomycin (Hospira) 14 days before sublethal irradiation and adoptive transfer. Naive CD8 + CD62L hi CD44 lo T cells (5 × 10 5 ) were stained with 5 μM CFSE and intravenously injected into the sub-lethally-irradiated, antibiotic-treated mice. At 8 days post transfer spleen and liver lymphocytes were stained with fluorochrome-conjugated α-CD8 and α-CD45.2 and analysed by flow cytometry. Quantification of bacterial 16S rDNA in mouse faeces Faecal pellets from antibiotic-treated and non-antibiotic-treated control mice were collected and snap-frozen in liquid nitrogen. DNA was isolated from faecal pellets with QIAamp DNA Stool Mini Kit (Qiagen, Germany) and quantified by UV spectrophotometry at 260 nm using the NanoDrop 1000 (Thermo Scientific). Degenerate primers for the V2 region of bacterial 16S DNA (forward: 5′-AGYGGCGIACGGGTGAGTAA-3′; reverse: 5′-CYIACTGCTGCCTCCCGTAG-3′) and primers for mouse pIgR genomic region (forward: 5′-TTTGCTCCTGGGCCTCCAAGTT-3′; reverse: 5′-AGCCCGTGACTGCCACAAATCA-3′) were designed as described [60] . PCR reactions were performed with 2 ng of DNA, Luminaris Color HiGreen qPCR Master Mix (Thermo Scientific) in a Rotor-Gene 3000 (Corbett) with a 15-min activation/denaturation step (95 °C); 40 cycles of 30 s denaturation (95 °C), 30 s annealing (60 °C) and 30 s extension (72 °C). The resulting PCR products were resolved on agarose gels and visualized by ethidium staining. Statistical analyses Statistical analyses were performed using the nonparametric, unpaired Mann–Whitney U- test or where indicated the one-way or two-way analysis of variance (ANOVA) test using Graphpad Prism software. P- values of <0.05 were considered significant. Outliers were removed with the ROUT-outlier test using Graphpad Prism software. How to cite this article: Wiede, F. et al . PTPN2 attenuates T-cell lymphopenia-induced proliferation. Nat. Commun. 5:3073 doi: 10.1038/ncomms4073 (2014).